GWAS meta-analysis of intrahepatic cholestasis of pregnancy implicates multiple hepatic genes and regulatory elements Intrahepatic cholestasis of pregnancy (ICP) is a pregnancy-specific liver disorder affecting 0.5–2% of pregnancies. The majority of cases present in the third trimester with pruritus, elevated serum bile acids and abnormal serum liver tests. ICP is associated with an increased risk of adverse outcomes, including spontaneous preterm birth and stillbirth. Whilst rare mutations affecting hepatobiliary transporters contribute to the aetiology of ICP, the role of common genetic variation in ICP has not been systematically characterised to date. Here, we perform genome-wide association studies (GWAS) and meta-analyses for ICP across three studies including 1138 cases and 153,642 controls. Eleven loci achieve genome-wide significance and have been further investigated and fine-mapped using functional genomics approaches. Our results pinpoint common sequence variation in liver-enriched genes and liver-specific cis -regulatory elements as contributing mechanisms to ICP susceptibility. Intrahepatic cholestasis of pregnancy (ICP) is a pregnancy-specific liver disorder affecting ~0.5–2% of pregnant women. The majority of cases present in the third trimester with pruritus. The diagnosis is confirmed by elevated maternal total serum bile acids (TSBA) and abnormal serum liver tests [1] . Elevation of maternal TSBA ≥40 µmol/L is associated with an increased incidence of adverse pregnancy outcomes [2] , [3] , and a large meta-analysis of ICP cases identified 100 µmol/L as the threshold at which the risk of stillbirth increases [4] . ICP has a complex etiology, with genetic, endocrine, and environmental contributions. A variable geographical prevalence has also been observed with this disease. This may be explained by genetic variation in women of different ancestry, or could be the result of altered environmental factors, e.g., vitamin D or selenium deficiency [5] . The cholestatic effect of gestational elevations of estrogen and progesterone metabolites unmasks the disease in genetically susceptible individuals [6] , [7] . Rare mutations in the hepatobiliary transporter genes ABCB4 and ABCB11 (encoding the phosphatidyl choline floppase and the bile salt export pump, respectively) have been reported, with the most recent study identifying pathogenic or likely pathogenic heterozygous mutations in either of these two genes in up to 25% of cases of severe, early-onset ICP [8] . A limited role has been proposed for rare genetic variants in other known cholestatic loci [9] . In contrast with rare variants, the contribution of common genetic variation to the heritability of ICP has not been systematically addressed thus far. Candidate gene analyses have been reported [10] but to date the only genome-wide study of ICP has employed admixture mapping of genetically distinct populations [11] . Here, we utilized the recent whole-genome sequencing study by the NIHR BioResource Rare Disease collaboration (NIHR-RD) and the 100,000 Genomes Project (100KGP) [12] along with data from the FinnGen Consortium to systematically identify common variants that contribute to ICP susceptibility. We have performed the first GWAS and meta-analyses for ICP, examining >7 million common sequence variants in 1138 cases of ICP compared to 153,642 non-ICP controls. This resulted in the identification of 11 genome-wide significant loci associated with ICP. The application of a functional prioritization pipeline further enabled the identification of liver-enriched genes and liver-specific cis -regulatory elements as likely effectors of ICP risk. GWAS and GWAS meta-analyses for ICP GWAS were first performed using the NIHR-RD ( https://bioresource.nihr.ac.uk/using-our-bioresource/our-cohorts/rare-diseases/ ) and 100KGP ( https://www.genomicsengland.co.uk/initiatives/100000-genomes-project ) data separately (Supplementary Fig. 1 ). In the NIHR-RD, 303 patients with ICP (severe, early-onset disease with symptoms by 33 weeks’ gestation and maternal TSBA ≥ 40 µmol/L) were recruited. For women that used hormonal contraception, 15/254 (5.9%) reported itching when used and 39/256 reported cyclical itching. In addition, 15/247 patients (6.1%) reported drug-induced itching (other than for contraception). In the 100KGP, 225 individuals with an International Classification of Diseases (ICD) code for ICP were identified across all 100KGP study cohorts. For each of these datasets, common (minor allele frequency (MAF) ≥0.01) high-quality variants were extracted from the whole-genome sequence data. An unrelated subset of individuals of genetically defined European (EUR) ancestry (Supplementary Fig. 2 ), was identified by kinship coefficient estimation and principal component analysis. After quality control, the NIHR-RD dataset comprised 216 cases and 8436 controls with 8,291,828 variants, and the 100KGP dataset comprised 182 cases and 45,585 controls with 9,429,238 variants. A GWAS was performed in each cohort separately using a generalized mixed model association test with saddle-point approximation to adjust for case–control imbalance using SAIGE [13] with sex and ten principal components (PCs) as covariates. The resulting summary statistics for variants with matching alleles and allele frequencies between the two datasets were then meta-analyzed using METAL [14] , weighting the effect size estimates using the inverse of the standard errors. Variants showing heterogeneity of effect between the two datasets ( P < 1 × 10 −5 ) were excluded. In total, 8,199,999 variants were meta-analyzed and four loci were identified as achieving genome-wide significance ( P < 5 × 10 −8 ) (Supplementary Figs. 1, 3a ). The genomic inflation (lambda) was 1.01 (Supplementary Fig. 3c ), indicating no significant population stratification. To enhance the power for genetic discovery, we meta-analyzed the NIHR-RD/100KGP (UK) ICP GWAS meta-analysis summary statistics with GWAS data from FinnGen (Release 4) ( https://www.finngen.fi/en ). FinnGen is a public-private partnership combining digital health record data from Finnish health registries with genotyping data from Finnish Biobanks. Release 4 includes association data at 16,962,023 variants for 2444 endpoints in 176,899 Finnish individuals. As with the 100KGP, cases of ICP were identified based on ICD codes. There were 740 cases and 99,621 controls following FinnGen phenotype evaluation. GWAS was performed by FinnGen using SAIGE [13] with sex, age, 10 PCs, and genotyping batch as covariates. Analysis of the summary statistics for the FinnGen ICP GWAS revealed seven loci achieving genome-wide significance (Supplementary Figs. 1, 3b, d ), including the four loci identified in the UK meta-analysis. After allele matching, allele frequency matching, and removal of heterogeneous effects, 7,715,762 variants were available for meta-analysis across all three cohorts. In total, 11 loci achieved the genome-wide significance threshold ( P < 5 × 10 −8 ), (Fig. 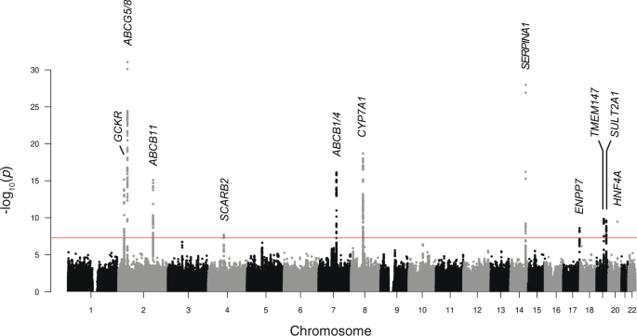Fig. 1: Manhattan plot for the genome-wide association study meta-analysis of intrahepatic cholestasis of pregnancy (ICP). Data shown are from the combined meta-analysis including 1138 cases and 153,642 controls, all of European ancestry. The chromosomes are ordered on thexaxis; theyaxis shows the −log10(P) values for the association tests. Eleven loci achieved genome-wide significance (P< 5 × 10−8, indicated by the red line). The prioritized gene at each locus is shown. The effector gene functional prioritization strategy followed in this study is presented in Fig.2. Association testing was performed using a generalized logistic mixed model to account for population stratification and saddle-point approximation to control for type 1 error rates due to unbalanced case–control ratios, followed by meta-analysis weighting the effect size estimates using the inverse of the standard errors. 1 , Table 1 , and Supplementary Fig. 1) and the genomic inflation (lambda) for the overall meta-analysis was 1.027 (Supplementary Fig. 3e ). Summary statistics for the lead variants in each of the separate GWAS and meta-analyses are provided in Supplementary Data 1 . Fig. 1: Manhattan plot for the genome-wide association study meta-analysis of intrahepatic cholestasis of pregnancy (ICP). Data shown are from the combined meta-analysis including 1138 cases and 153,642 controls, all of European ancestry. The chromosomes are ordered on the x axis; the y axis shows the −log 10 ( P ) values for the association tests. Eleven loci achieved genome-wide significance ( P < 5 × 10 −8 , indicated by the red line). The prioritized gene at each locus is shown. The effector gene functional prioritization strategy followed in this study is presented in Fig. 2 . Association testing was performed using a generalized logistic mixed model to account for population stratification and saddle-point approximation to control for type 1 error rates due to unbalanced case–control ratios, followed by meta-analysis weighting the effect size estimates using the inverse of the standard errors. Full size image Table 1 Association statistics of the eleven loci achieving genome-wide significance ( P < 5 × 10 −8 ) in the genome-wide association study meta-analysis of intrahepatic cholestasis of pregnancy (ICP). Full size table Conditional and joint (GCTA-COJO) [15] analyses in each of the genome-wide significant loci demonstrated a single signal underlying each association. Testing for epistatic interactions was performed across all 55 possible pairs of the 11 risk variants in NIHR-RD and 100KGP (for which full genotype data were available) separately with PLINK [16] and the resulting P values were combined using Fisher’s method. No significant interactions were identified after correcting for multiple testing based on 55 comparisons ( P < 0.0009). Post hoc power calculations based on the size of the cohort utilized for the combined meta-analysis demonstrated 80% power to detect effects with an odds ratio (OR) > 1.3 at MAF = 0.5 and OR > 1.7 at MAF ≥ 0.05 (Supplementary Fig. 4 ). Functional fine-mapping of causal variants at ICP susceptibility loci The liver is a central organ in the development of ICP, as evidenced by the fact that most known ICP causal mutations affect liver-specific genes [8] , [9] (Supplementary Fig. 5a ). Moreover, unbiased analysis of the 11 ICP association signals from our GWAS highlighted that the expression of genes within these loci is highly liver-specific (Supplementary Fig. 5b ) and relate to pathways involved in bile acid and lipid metabolism (Supplementary Fig. 6 ). We, therefore, reasoned that both coding and noncoding ICP risk variants likely affect liver-specific genes and/or cis -regulatory elements (CREs). In order to gain insights into the genetic mechanisms driving ICP susceptibility and identify likely causal variants, we carried out functional fine-mapping of the 11 association signals detected in the meta-analysis using PAINTOR [17] to calculate the probability of a variant being causal at a given locus considering not only its strength of association but also functional annotation data (Fig. 2 ). We included adult liver tissue active chromatin features in the datasets used to prioritize causal variants, including accessible chromatin regions and those enriched in H3K27ac (see “Methods”). This analysis enabled the prioritization of nine variants with a high functional posterior probability (PP func > 0.8) across eight ICP susceptibility loci (Supplementary Data 2 ). For the remaining three loci, which did not include any protein-altering variant, we assumed that variants residing within active liver CREs were more likely functional. 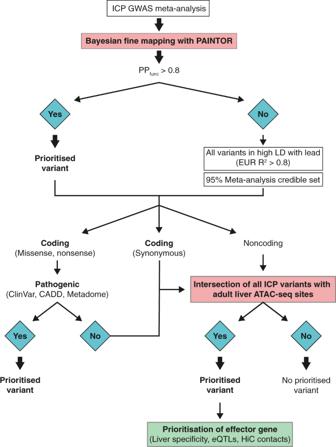Fig. 2: Flowchart describing the variant prioritization strategy followed for the eleven loci reaching genome-wide significance in the GWAS meta-analysis of ICP. Sequential steps used to prioritize the variants are shown with the different approaches for nonsynonymous, synonymous, and noncoding variants indicated. We thus defined a high-confidence set of human liver accessible chromatin sites using ATAC-seq profiles from four whole liver samples (data from ENCODE [18] , see “Methods”), which allowed us to further prioritize one likely causal variant at each remaining locus (Table 2 ). Fig. 2: Flowchart describing the variant prioritization strategy followed for the eleven loci reaching genome-wide significance in the GWAS meta-analysis of ICP. Sequential steps used to prioritize the variants are shown with the different approaches for nonsynonymous, synonymous, and noncoding variants indicated. Full size image Table 2 Prioritized variants and genes within each of the eleven ICP genome-wide significant loci. Full size table ICP coding variant analysis Three ICP signals ( SERPINA1 , GCKR , and HNF4A ) hosted a single missense coding variant with high likelihood of being causal, with functional posterior probabilities above 99% and a pathogenicity score CADD >10 [19] (Fig. 3 ). From these three signals, the one with the strongest association with ICP susceptibility was rs28929474 in the SERPINA1 gene, which encodes alpha-1-antitrypsin, a major plasma serine protease inhibitor (Fig. 3a ). This variant has been extensively reported in the literature as the SERPINA1 Z allele, an amino acid substitution of Glu342Lys that causes alpha-1-antitrypsin deficiency [20] and is associated with cystic fibrosis liver disease [21] . The two other missense variants alter the sequences of the GCKR (glucokinase regulatory protein) and HNF4A (hepatic nuclear factor 4 alpha) (Fig. 3b, c ), genes that are essential for hepatic metabolic homeostasis and when mutated may lead to monogenic diabetes [22] . We examined the potential functional impact of these coding variants through the querying of the ClinVar variant interpretation database and Metadome analysis [23] . At GCKR , we identified an ICP risk variant, rs1260326 (Leu446Pro), which has been previously associated with altered serum fasting plasma glucose and triglyceride concentrations [24] , [25] and nonalcoholic fatty liver disease (NAFLD) [26] . Previous functional studies of this variant have indicated that the risk allele in this locus is associated with increased glucokinase activity in the liver [27] . At HNF4A , a single variant was associated with ICP susceptibility, rs1800961 (Thr139Ile), which Metadome analysis [23] predicted to be deleterious for protein function (Supplementary Fig. 7a ). Fig. 3: Analysis of intrahepatic cholestasis of pregnancy (ICP) association signals uncovers three coding risk variants affecting the SERPINA1 , GCKR , and HNF4A genes. a – c Regional association and linkage disequilibrium (LD) plots for the ICP signals at SERPINA1 , GCKR , and HNF4A , respectively. The y axis represents the −log 10 ( P ) values for the association test from the GWAS meta-analysis of ICP (1138 cases and 153,642 controls) and the x axis the chromosomal positions (GRCh38/hg38). The SNP with the lowest p-value in the locus is indicated by a purple diamond. The remaining SNPs in the region are colored according to their r 2 with the lead SNP ( r 2 calculated using 1000 Genomes European (EUR) reference). The dotted gray line represents the genome-wide significance threshold of 5 × 10 −8 . Plots were generated using LocusZoom [61] . Association testing was performed as described in Fig. 1 . Zoomed insets reveal the prioritized coding variant at each locus, with functional posterior probability (PP func ) above 0.99. PP func were calculated using PAINTOR [17] . All three variants showed Combined Annotation Dependent Depletion (CADD) scores [19] , [84] above 10, which is usually considered the threshold for pathogenic variants. Further details on coding variant analysis are provided in Supplementary Data 3 . 95% PP ICP variants, variants within the 95% genetic credible set in the ICP meta-analysis. LD ICP variants, variants with EUR r 2 > 0.8 with the meta-analysis lead variant. Full size image Functional prioritization of noncoding variants at lipid and bile acid homeostasis loci At the remaining loci identified in the GWAS meta-analysis for ICP, we observed that seven of the eleven loci contained noncoding and synonymous variants (examining the 95% genetic credible set, as well as the lead variant and those in linkage equilibrium at r 2 > 0.8 in EUR individuals). This observation is in line with previous reports suggesting that common sequence variation predominantly contributes to human disease via disruption of noncoding cis -regulatory elements [28] , [29] . We therefore took advantage of the functional fine-mapping strategy described above, along with the integration of adult liver epigenomic datasets and pathogenicity measures, to further dissect the causal mechanisms at play in each ICP locus (Fig. 2 , see “Methods”). In the liver, the family of ABC transporters play central roles in numerous physiological processes, including the export of cholesterol, bile salts, bilirubin, and drug conjugates. Three ABC transporter gene loci ( ABCG5/8 , ABCB1/4 , and ABCB11 ) contained ICP GWAS signals (Fig. 4 ). ABCG5 and ABCG8 together encode a heterodimeric cholesterol transporter, expressed in hepatocytes and intestinal cells [30] . A missense polymorphism in ABCG8 , Tyr54Cys (rs4148211), was identified as the lead variant at this locus (Fig. 4a ). However, Metadome analysis [23] indicated that this protein sequence change is expected to be tolerated (Supplementary Fig. 7b and Supplementary Data 3 ), suggesting that this or other variants in linkage disequilibrium (LD) have a different type of functional impact at this locus. Combined analysis of adult liver epigenomic datasets and a high-throughput reporter assay dataset from liver cells (Survey of Regulatory Elements, SuRE [31] ), indicated that the lead variant rs4148211 (PP func > 0.99) resides within a hepatic CRE and its risk allele is associated with allele-dependant transcriptional activity in liver cells ( P = 9.1 × 10 −4 ), where the risk allele is associated with transcriptional repression (Fig. 4b and Supplementary Fig. 7c ). Analysis of the SuRE assay dataset from liver cells revealed seven additional ICP-associated variants in the ABCG8 locus for which the risk allele associates with transcriptional repression (Supplementary Fig. 7c ). However, only one overlapped a hepatic CRE (rs4148204) and none of them was prioritized as likely causal by PAINTOR (Supplementary Data 2 ). Fig. 4: Three ABC transporter gene loci are associated with intrahepatic cholestasis of pregnancy (ICP). a , c , e LocusZoom [61] plots showing the association signals at ABCG8 , ABCB1/4 , and DHRS9 , respectively. The LocusZoom plots are as per Fig. 3 and association testing was performed as described in Fig. 1 . At each locus, a single noncoding variant was prioritized as likely causal following the strategy outlined in Fig. 2 . All epigenomic and transcriptomic datasets shown were retrieved from ENCODE [18] . Adult liver ATAC-seq peaks track (green regions) corresponds to regions accessible in at least two out of four ENCODE adult liver ATAC-seq (see Methods). 95% PP ICP variants, variants within the 95% genetic credible set in the ICP meta-analysis. LD ICP variants, variants with EUR r 2 > 0.8 with the meta-analysis lead variant. PP func , functional posterior probability calculated using PAINTOR [17] . CADD, combined annotation-dependent depletion. a Zoomed inset shows a coding variant at ABCG8 overlapping a hepatic transcriptional enhancer, as revealed by strong H3K27ac enrichment and accessible chromatin in adult female liver tissue. Metadome analysis did not suggest that this variant affects protein function (see Supplementary Fig. 7 ). b Allele-specific effect of the prioritized risk variant rs4148211, assessed by Survey of Regulatory Elements (SuRE) in HepG2 cells [31] . The results suggest that the risk variant associates with decreased transcriptional activity. Mean signal and two-sided Wilcoxon rank-sum test. Previously determined 5% false-discovery rate threshold: P < 0.00173121 [31] . Source data are provided as a Source Data file. c , e Zoomed insets show two prioritized regulatory risk variants for ICP: one affecting a hepatic enhancer between ABCB1 and ABCB4 ( c ), and one affecting a hepatic enhancer in an intron of DHRS9 ( d ). We note however that DHRS9 is not expressed in liver tissue, as shown in the strand-specific RNA-seq tracks. In contrast, ABCB11 is highly expressed in this tissue making it a likely effector transcript in this locus. Full size image The ICP association signal on chromosome 7 spanned a genomic segment including the genes ABCB1 and ABCB4 (Fig. 4c ), which encode for the Multidrug Resistance Proteins 1 and 3 (MDR1 and MDR3), respectively. Whilst the lead variant in this locus did not overlap a coding sequence or active hepatic CRE, we prioritized the variant rs55747905 as likely functional (PP func = 0.94), which overlapped an active enhancer element (accessible chromatin enriched in H3K27ac) (Fig. 4c ). Transcription factor binding motif disruption analysis further revealed that the risk allele of rs55747905 (C) disrupts a recognition sequence for the Wnt signaling transcription factor TCF7L2 (Fig. 4d ). At the third ABC transporter locus, we prioritized ABCB11 as the gene mediating the ICP susceptibility process. In this case, functional fine-mapping with PAINTOR enabled the prioritization of a single variant residing in an intronic liver enhancer in the DHRS9 gene (Fig. 4e ). However, analysis of ENCODE [18] RNA-seq data revealed that DHRS9 has very weak expression in adult liver, in contrast with ABCB11 , which encodes the bile salt export pump (BSEP). The ICP association signal on chromosome 8 is located between the UBXN2A and CYP7A1 genes (Fig. 5a ). UBXN2A encodes a ubiquitin-like protein involved in proteasomal degradation [32] and CYP7A1 encodes the enzyme (cholesterol 7 alpha-hydroxylase) responsible for the first and rate-limiting step in bile acid biosynthesis in hepatocytes [33] . At this locus, only one regulatory variant was prioritized, rs10504255, which resides in an active liver enhancer. Unlike the lead variant at this locus (rs10107182), the prioritized variant reached a high functional posterior probability (PP func > 0.99 vs. <0.01) and had a high pathogenicity score (CADD = 12.9 vs. 5.8). Furthermore, analysis of GTEx [34] eQTL data revealed that rs10504255 is associated with allele-dependant expression of UBXN2B in human liver (Fig. 5b ), where the risk allele (G) is associated with weaker transcriptional activity ( P = 6.18 × 10 −6 ). Even though this variant was not a statistically significant eQTL for CYP7A1 in the GTEx database ( P = 0.15), we observed a similar trend on the direction of effect of the risk allele (Fig. 5b ) and previous chromatin conformation capture and genome editing studies in human hepatocytes have linked this CRE with the modulation of CYP7A1 expression [35] . These previous studies, combined with the functional significance of CYP7A1 in bile acid homeostasis, led us to prioritize CYP7A1 as the major effector transcript in this locus. Motif analysis further revealed that the risk allele disrupts a binding site for the transcription factor DMRTA1 (Fig. 5c ). Fig. 5: GWAS meta-analysis of ICP reveals association signals affecting the bile acid homeostasis genes CYP7A1 and SULT2A1 . a , d LocusZoom [61] plots showing the association signals at CYP7A1 and SULT2A1 , respectively. The LocusZoom plots are as per Fig. 3 and association testing was performed as described in Fig. 1 . All epigenomic and transcriptomic datasets shown were retrieved from ENCODE [18] . Adult liver ATAC-seq peaks track (green regions) corresponds to regions accessible in at least two out of four ENCODE adult liver ATAC-seq (see “Methods”). 95% PP ICP variants, variants within the 95% genetic credible set in the ICP meta-analysis. LD ICP variants, variants with EUR r 2 > 0.8 with the meta-analysis lead variant. PP func , functional posterior probability calculated using PAINTOR. CADD, combined annotation-dependent depletion. a Functional fine-mapping with PAINTOR [17] identified a single variant (rs10504255) with a posterior probability over 0.99 overlapping an active liver enhancer located between the CYP7A1 gene, which encodes the rate-limiting enzyme for bile acid synthesis, and UBXN2B . b , e GTEx [34] [GTEx Analysis Release V8 (dbGaP Accession phs000424.v8.p2)] human liver eQTLs identify the top prioritized variant in the CYP7A1 locus (rs10504255) as an eQTL associated with the eGene UBXN2B ( b ) and show that the SULT2A1 promoter ICP variant (rs296361) is an eQTL for both SULT2A1 and its downstream lncRNA LINC01595 ( e ). Violin plots represent the density distribution of the samples in each genotype ( n for each genotype is indicated below in blue). Box plots show normalized gene expression in median (white line), first and third quartiles. Gene-level adjusted P values calculated with FastQTL [85] are shown. c The risk allele of the ICP-associated variant rs10504255 (G) disrupts a DMRTA1-binding motif. We note that this allele also associates with weaker transactivation in liver tissue, as observed by eQTL analysis ( b ). d Overlap of ICP risk variants with adult liver accessible chromatin sites revealed one variant in the promoter of SULT2A1 (rs296361). f Transcription factor motif analysis revealed that the ICP variant rs296361 affects a motif for the SOX-D transcriptional repressor family. Full size image In addition to CYP7A1 , the ICP GWAS meta-analysis identified another important locus for bile acid homeostasis, SULT2A1 , which encodes the enzyme Sulfotransferase 2A1, highly expressed in the liver and capable of phase II metabolism of bile acids [36] (Fig. 5d ). Here, a variant in the promoter of SULT2A1 was prioritized (rs296361), with the risk allele conferring lower SULT2A1 expression in the liver ( P = 1.31 × 10 −7 ) (Fig. 5e ), likely through the creation of a binding site for the family of transcriptional repressors SOX-D (Fig. 5f ). We note that the prioritized variant also associated with allele-dependent effects on the expression of a nearby long noncoding RNA ( LINC01595 , P = 1.02 × 10 −50 ), albeit in the opposite direction. This discrepancy may reflect an indirect effect of the expression of SULT2A1 on LINC01595 . Functional prioritization of previously uncharacterized ICP genes We next explored the remaining three ICP-associated signals where the closest genes were not directly involved in lipid and bile acid homeostasis. On chromosome 19, even though it was not possible to employ PAINTOR for functional fine-mapping due to the presence of ambiguous alleles (A/T or G/C), we prioritized the variant rs4806173 based on its overlap with a hepatic CRE (Fig. 6a ). This variant resides in an intron of the testis-specific gene GAPDHS [37] . We thus queried eQTL GTEx [34] data to identify potential targets of this regulatory variant in liver tissue. This analysis led us to pinpoint TMEM147 (transmembrane protein 147) as the likely effector transcript of this association signal, with the risk allele associating with lower hepatic gene expression (1.52 × 10 −40 ) (Fig. 6b ). Using transcription factor motif disruption analysis, we detected that the risk allele of rs4806173 creates a recognition sequence for the glucocorticoid receptor (Fig. 6c ), which has been previously reported to act as either a gene expression activator or repressor in a context-dependent manner [38] , [39] . Recent studies in HeLa cells have linked loss of TMEM147 with increased cholesterol uptake [40] supporting the role of this gene as an effector of ICP genetic susceptibility. Fig. 6: Analysis human liver eQTLs uncovers TMEM147 and ENPP7 as effector transcripts of ICP susceptibility. a , d LocusZoom [86] plots showing the association signals at TMEM147 and ENPP7 , respectively. The LocusZoom plots are as per Fig. 3 and association testing was performed as described in Fig. 1 . All epigenomic and transcriptomic datasets shown were retrieved from ENCODE [18] . Adult liver ATAC-seq peaks track (green regions) corresponds to regions accessible in at least two out of four ENCODE adult liver ATAC-seq (see “Methods”). 95% PP ICP variants, variants within the 95% genetic credible set in the ICP meta-analysis. LD ICP variants, variants with EUR r 2 > 0.8 with the meta-analysis lead variant. PP func , functional posterior probability calculated using PAINTOR [17] . CADD, combined annotation-dependent depletion. Overlap of ICP-associated variants in these two loci with adult liver accessible chromatin sites enabled the prioritization of two ICP regulatory variants in intronic regions of GAPDHS (rs4806173) ( a ) and ENPP7 (rs9916601) ( d ). b , e The ICP variants prioritized with functional liver chromatin annotations are eQTLs in liver tissue and pinpoint TMEM147 and ENPP7 as effector transcripts in these loci. Violin plots represent the density distribution of the samples in each genotype ( n for each genotype is indicated below in blue). Box plots show normalized gene expression in median (white line), first and third quartiles. Gene-level adjusted P values calculated with FastQTL [86] are shown. Liver eQTL plots were retrieved from GTEx [34] [GTEx Analysis Release V8 (dbGaP Accession phs000424.v8.p2)]. We note that GAPDHS is a testis-specific gene and its interrogation as an eGene for rs4806173 was therefore not possible ( b ). c The ICP risk allele of rs4806173 (G), which associates with less transcription of TMEM147 , is predicted to create a binding site for glucocorticoid receptors, a family of context-dependent transcriptional regulators that can act as either activators or repressors [87] . Full size image Similarly, we prioritized ENPP7 as the likely effector transcript driving the association signal in chromosome 17 (Fig. 6d, e ), with the risk variant (T) associating with increased ENPP7 expression (Fig. 5e ). ENPP7 encodes the alkaline sphingomyelinase (Alk-SMase) that is present in the intestinal tract and bile, and responsible for the digestion of sphingomyelins in a bile salt-dependent manner [41] . Previous studies have suggested that Alk-SMase promotes intestinal cholesterol absorption [42] . The final signal encompassed intronic variants in the SHROOM3 gene, including one variant in a hepatic CRE (rs4859682) (Fig. 7a ). However, analysis of liver eQTLs did not assist in the identification of potential effector transcripts in the locus. Topologically associating domains (TADs) correspond to self-interacting genomic domains that contain genes and regulatory elements that interact more frequently with each other than with other regions [43] . We thus carried out a systematic analysis of all genes located in the TAD that contains this ICP association signal, interrogating their expression in liver tissue (Fig. 7b) and their liver-specificity (Fig. 7c ). Given the liver-specificity of most ICP genes (Supplementary Fig. 5b ), we decided to further investigate genes whose expression is both high and specific in liver tissue. Two genes met these criteria: STBD1 and SCARB2 (Fig. 7c ). We then investigated human liver Hi-C maps in order to find out whether there were long-range 3D chromatin contacts between the prioritized causal variant rs4859682, SHROOM3 (closest gene), STBD1, and SCARB2 , in this tissue. Only long-range interactions stemming from SCARB2 were detected (Fig. 7d ), which led us to prioritize this gene as the likely effector of the association signal in this locus. SCARB2 encodes for the lysosomal integral membrane protein type 2 (LIMP-2), which has been reported to play a role in cholesterol transport in lysosomes [44] . Fig. 7: Tissue-specificity and 3D chromatin conformation analyses prioritize SCARB2 as an ICP susceptibility gene. a LocusZoom [86] plot showing the association signal at SHROOM3 . The LocusZoom plots are as per Fig. 3 and association testing was performed as described in Fig. 1 . All epigenomic and transcriptomic datasets shown were retrieved from ENCODE [18] . Adult liver ATAC-seq peaks track (green regions) corresponds to regions accessible in at least two out of four ENCODE adult liver ATAC-seq (see “Methods”). 95% PP ICP variants, variants within the 95% genetic credible set in the ICP meta-analysis. LD ICP variants, variants with EUR r 2 > 0.8 with the meta-analysis lead variant. CADD, combined annotation-dependent depletion. Overlap of ICP risk variants in this locus with adult liver accessible chromatin sites enabled the prioritization of a single ICP-regulatory variant in an intronic region of the SHROOM3 gene (rs4859682). None of the other ICP variants (EUR r 2 > 0.8 with lead variant or in the 95% PP credible set) overlapped accessible chromatin sites. b Expression of all genes within the TAD containing the ICP lead variant rs13146355 in the human liver. Expression data was retrieved from GTEx [34] [GTEx Analysis Release V8 (dbGaP Accession phs000424.v8.p2)]. Violin plots represent the density distribution of expression of the indicated genes in human liver tissue ( n = 226 donors). Box plots show gene expression in median (white line), first and third quartiles. TPM, transcripts per million. Note that the gene harboring the ICP risk variant, SHROOM3 , is lowly expressed in the liver. c Scatter plot showing the expression of all genes within the TAD containing the ICP lead variant rs13146355 in the human liver versus their liver-specificity. Tissue-specificity scores (SPECS) were precalculated by Everaert et al. [81] . Source data are provided as a Source Data file. This plot highlights two highly expressed and liver-specific genes, STBD1, and SCARB2 . d , Analysis of long-range chromatin interactions in human liver detected by promoter capture Hi-C [79] , showing that the genomic region containing the ICP risk variant rs4859682 interacts with SCARB2 , but not SHROOM3 . Long-range chromatin interactions stemming from the promoter of STBD1 were not detected in liver tissue. Full size image Overlap of risk loci for ICP and other traits All but one of the loci identified in this study (rs34491636, ENPP7 ) have been previously associated (at r 2 > 0.6) with diseases or traits in the GWAS Catalog [45] , many of which have phenotypic overlap with ICP (Supplementary Fig. 8 and Supplementary Data 4 ). Notably, six of the loci have previously been associated with gallstone disease, six with LDL cholesterol concentrations, and four with liver enzyme concentrations (Supplementary Fig. 8 ). Likewise, we observed a strong enrichment for ICP susceptibility genes (identified in an unbiased manner from the GWAS loci) being also associated with gallstone disease ( P = 2.5 × 10 −15 ) and LDL cholesterol ( P = 2.67 × 10 −07 ) (Supplementary Fig. 9 ). The elevated serum bile acids that form the core phenotype are also associated with maternal and fetal dyslipidemia [46] , [47] , [48] , and increased rates of gallstone formation [49] . Variation at ABCG8 has previously been linked to gallstone disease and other lipid-related phenotypes [50] , [51] . However, the specific haplotype associated with ICP differs from the main reported association with gallstone disease. CYP7A1 variation is associated with blood lipid traits [52] in addition to gallstone formation [53] . Heterozygous ABCB4 mutations were the first genetic link identified to ICP [54] , [55] and common variation at this locus has been previously described in ICP [10] . In the context of pregnancy, raised gestational hormones cause reduced FXR-mediated induction of hepatic Bsep, Shp, and Mdr3 [6] , and enterocyte Shp and Fgf15/19 [56] thereby causing abnormal bile acid homeostasis. This is likely to exacerbate susceptibility to hypercholanemia in genetically predisposed women with the variants reported in this manuscript. Given the strong overlap between genes associated with ICP and cholelithiasis (Supplementary Fig. 9 ), we directly examined the evidence of association of the 11 ICP loci with cholelithiasis using the FinnGen cholelithiasis GWAS ( https://r4.finngen.fi/pheno/K11_CHOLELITH ), which includes 15,683 cases and 158,425 controls. Six of the loci identified in our ICP GWAS meta-analysis achieve genome-wide significance for cholelithiasis as well ( P < 5 × 10 −08 ) (Supplementary Fig. 8 ). Two additional loci demonstrate nominal evidence of association. Despite 100% power (assuming a similar-sized effect on the risk of ICP and cholelithiasis) to detect association, three ICP loci ( ABCB11 , SCARB2 , and ENPP7 ) showed no evidence of association with cholelithiasis indicating that they are specific to ICP and not shared with cholelithiasis. We also directly examined evidence of association at the 29 loci with AF > 0.01 (the MAF threshold in our study) previously associated with cholelithiasis in the largest meta-analysis published to date (comprising 27,174 cholelithiasis cases and 736,838 controls [57] ). Five of these loci achieve genome-wide significance ( P < 5 × 10 −08 ) in the ICP meta-analysis ( SERPINA1 , CYP7A1 , GCKR , ABCB4, and HNF4A ) and a further five show evidence of association with ICP after correcting for examining 29 loci ( P < 0.05/29 = 0.0017); two of these are genes reported as genome-wide significant in the present ICP GWAS ( ABCG8 and SULT2A1 ) and three are not ( FADS2 , JMJD1C , and TTC39B ). Assuming the same effect size of these associations between cholelithiasis and ICP, the power to detect association at P = 0.0017 was only present for one locus (at which significance was achieved) so we examined whether a composite effect of the known cholelithiasis genetic risk variants was detectable in ICP patients by calculating polygenic risk scores (PRS). Of the 29 cholelithiasis loci, genotype data were available in the NIHR-RD dataset for 27. PRS calculated using the OR from the previously published cholelithiasis GWAS demonstrated ICP patients have a significantly higher burden of cholelithiasis genetic risk variants compared with controls (Wilcoxon P = 1.4 × 10 −05 ). However, when this analysis was repeated with the above loci that showed association in the ICP meta-analysis removed (leaving 18 variants for which data were available), there was no difference in PRS ( P = 0.198) between ICP and controls, despite 92% power to detect a difference at P < 0.05. This suggests that not all the genetic risk factors for cholelithiasis are risk factors for ICP. Together, these findings indicate that cholelithiasis and ICP have distinct but overlapping sets of genetic risk factors. Given the overlapping genetic architecture between ICP and gallstone disease, and the broad spectrum of disease severity in this group, these loci represent possible modifier genes in a number of other cholestatic diseases such as the progressive familial cholestasis syndromes [58] . In conclusion, this study has uncovered common variation that influences ICP susceptibility, identifying key contributing genes. These genes highlight an underlying shared mechanism of variation at liver-specific genes and cis -regulatory elements, providing insights into the pathogenesis of this disease that warrant further investigation. Study cohorts and ethics An extensive description of the cohorts included in this study and details of the ethics approvals can be found in the Supplementary Note in Methods (Supplementary Information). NIHR-RD and 100KGP whole-genome sequencing variant calling, quality control, ancestry, and relatedness estimation Detailed methods describing the processing of whole-genome sequence data for the NIHR-RD and 100KGP cohorts can be found in the Supplementary Note in Methods (Supplementary Information). NIHR-RD and 100KGP genome-wide association analyses For genome-wide association analysis (GWAS) in both the NIHR-RD and 100KGP cohorts separately, variants passing the following criteria were retained: MAF ≥ 0.01, minimum minor allele count (MAC) ≥ 20, missingness <1%, Hardy–Weinberg equilibrium P value >1 × 10 −6 and differential (case/control) missingness P value >1 × 10 −5 . The final NIHR-RD and 100KGP datasets comprised 8,337,027 and 9,545,879 variants, respectively. GWAS was performed in each dataset separately using the R package SAIGE [13] (versions 0.42.1 and 0.44.2) ( https://github.com/weizhouUMICH/SAIGE ). SAIGE implements a generalized logistic mixed model to account for population stratification and a saddle-point approximation to control type 1 error rates when case–control ratios are unbalanced. SAIGE was run using the default parameters. Null logistic mixed models were fitted using the subsets of linkage disequilibrium (LD)-free high-quality common SNVs. Sex and the top ten principal components were used as fixed effects. The genomic inflation factors (lambda), calculated based on the 50th percentile, were 1.009 and 1.001 in NIHR-RD and 100KGP, respectively, indicating no evidence of confounding by population structure. The summary statistics from the NIHR-RD were lifted over from build GRCh37 to build GRCh38 of the human genome using CrossMap [59] (version 0.5.2) ( http://crossmap.sourceforge.net/ ). In all, 12,756 variants failed to lift over. Due to data sharing restrictions, it was not possible to combine the raw genome-wide genotype data from the NIHR-RD and 100KGP datasets. NIHR-RD and 100KGP meta-analysis Meta-analysis of the NIHR-RD and 100KGP GWAS summary statistics was performed using METAL (version 2011-03-25) ( https://genome.sph.umich.edu/wiki/METAL ) [14] . Multi-allelic variants were excluded such that there were 8,291,828 and 9,545,879 variants in NIHR-RD and 100KGP, respectively. Of these, 8,207,819 variants were shared and 8,201,630 variants had matching alleles. Meta-analysis was performed weighting the effect size estimates using the inverse of the standard errors. Variants showing heterogeneity of effect between the two datasets ( P < 1 × 10 −5 ) and those in which the minimum/maximum allele frequencies differed by >0.05 were excluded leaving 8,199,999 variants. 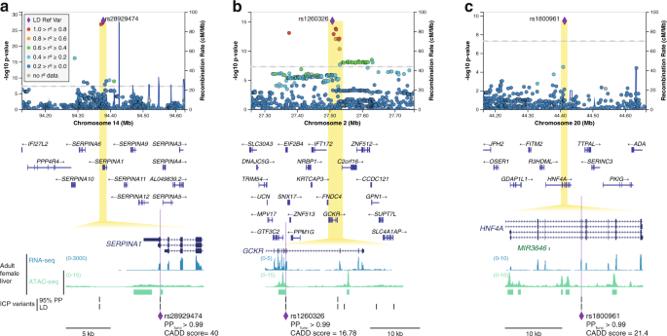Fig. 3: Analysis of intrahepatic cholestasis of pregnancy (ICP) association signals uncovers three coding risk variants affecting theSERPINA1,GCKR, andHNF4Agenes. a–cRegional association and linkage disequilibrium (LD) plots for the ICP signals atSERPINA1,GCKR, andHNF4A, respectively. Theyaxis represents the −log10(P) values for the association test from the GWAS meta-analysis of ICP (1138 cases and 153,642 controls) and thexaxis the chromosomal positions (GRCh38/hg38). The SNP with the lowest p-value in the locus is indicated by a purple diamond. The remaining SNPs in the region are colored according to theirr2with the lead SNP (r2calculated using 1000 Genomes European (EUR) reference). The dotted gray line represents the genome-wide significance threshold of 5 × 10−8. Plots were generated using LocusZoom61. Association testing was performed as described in Fig.1. Zoomed insets reveal the prioritized coding variant at each locus, with functional posterior probability (PPfunc) above 0.99. PPfuncwere calculated using PAINTOR17. All three variants showed Combined Annotation Dependent Depletion (CADD) scores19,84above 10, which is usually considered the threshold for pathogenic variants. Further details on coding variant analysis are provided in Supplementary Data3. 95% PP ICP variants, variants within the 95% genetic credible set in the ICP meta-analysis. LD ICP variants, variants with EURr2> 0.8 with the meta-analysis lead variant. A Manhattan plot was produced using the R package qqman (version 0.1.8) ( https://github.com/stephenturner/qqman ) [60] (Supplementary Figure 3a ). Four loci achieved genome-wide significance ( P < 5 × 10 −8 ). A QQ plot was generated using the observed and expected –log10 ( P values) (Supplementary Fig. 3c ). The genomic inflation factor (lambda), calculated based on the 50th percentile, was 1.01 indicating no significant population stratification. FinnGen genome-wide association analysis FinnGen is a public-private partnership combining digital health record data from Finnish health registries with genotyping data from Finnish Biobanks. Release 4 ( https://finngen.gitbook.io/documentation/v/r4/ ) includes association data at 16,962,023 variants for 2444 endpoints in 176,899 Finnish individuals. A detailed description of the study design and analytical methods are available in the online documentation (URL above). In brief, individuals were genotyped with Illumina and Affymetrix chip arrays. QC was performed to remove samples and variants of poor quality. Genome-wide imputation was performed using reference Finnish whole-genome sequence data. Disease endpoints were defined using nationwide registries based on ICD (and other) codes. A subset of unrelated individuals of genetically confirmed Finnish ancestry was identified. GWAS was performed using SAIGE (version 0.35.8.8) for all variants with MAC > 5. Sex, age, 10 PCs, and genotyping batch were included as covariates in the analysis. For the ICP GWAS ( https://r4.finngen.fi/pheno/O15_ICP ), cases ( n = 740) were identified as those with the ICD-10 code of O26.6 (“Liver disorders in pregnancy, childbirth and the puerperium” including “cholestasis (intrahepatic) in pregnancy” and “obstetric cholestasis”) or an ICD-9 code of 646.7 (“Liver and biliary tract disorders in pregnancy”). All females without these ICD codes were included as controls ( n = 99,621). Seven loci achieved genome-wide significance ( P < 5 × 10 −8 ) (Supplementary Fig. 3b ). The genomic inflation factor (lambda), calculated based on the 50th percentile, was 1.046 (Supplementary Fig. 3d ). Combined UK (NIHR-RD and 100KGP) and FinnGen meta-analysis A meta-analysis was subsequently performed of the combined NIHR-RD and 100KGP data (“UK meta-analysis”) and the FinnGen summary statistics. This included 154,780 individuals of whom 1138 were cases and 153,642 were controls. Meta-analysis was performed using the same methodology as described above. A total of 7,721,597 variants were shared between the final UK meta-analysis dataset and the FinnGen dataset and 7,715,997 variants had matching alleles. After performing the meta-analysis, variants showing heterogeneity of effect between the two datasets ( P < 1 × 10 −5 ) and those in which the minimum/maximum allele frequencies differed by >0.25 were excluded leaving 7,715,762 variants. Eleven loci achieved genome-wide significance ( P < 5 × 10 −8 ) (Fig. 1 ). The genomic inflation factor (lambda), calculated based on the 50th percentile, was 1.027 (Supplementary Fig. 3e ). Summary statistics for each of the lead variants in each of the separate GWAS and meta-analyses are provided in Supplementary Data 1 . LocusZoom Regional high-resolution association plots showing the LD between markers in the prioritized loci (as per European reference data) were generated using LocusZoom (version 0.13.3) ( https://my.locuszoom.org/ ) [61] . Credible sets were calculated by LocusZoom using Bayes factors based on the P values ( https://statgen.github.io/gwas-credible-sets/method/locuszoom-credible-sets.pdf ). Epistasis Testing for epistatic interactions was performed across all possible 55 pairs of the 11 prioritized lead risk variants in NIHR-RD and 100KGP separately with PLINK [16] (version 1.9) ( https://www.cog-genomics.org/plink/ ). The resulting P values were combined using Fisher’s method. No significant interactions were identified after correcting for multiple testing based on 55 comparisons ( P < 0.0009). Conditional analysis Each of the prioritized loci was examined using “conditional and joint analyses” (GCTA-COJO) [15] to assess whether there was more than one independent signal. COJO was run from GCTA (version 1.93.2) ( https://cnsgenomics.com/software/gcta/#COJO ) using default parameters (examining a 10-Mb window surrounding genome-wide significant variants). The NIHR-RD dataset was utilized to provide the reference LD structure of the variants. Power calculations Post hoc power calculations were performed to assess the range of odds ratio (OR) and allele frequencies for which associations could be detected at genome-wide significance ( P < 5 × 10 −8 ) given the number of cases and controls in the final meta-analysis. The R package genpwr [62] (version 1.0.4) ( https://cran.r-project.org/web/packages/genpwr/index.html ) was employed using a logistic model under genetic additivity. Power to detect specific previously described associations was calculated with genpwr using the OR of the described associations, reference European AF and cohort sizes. For cholelithiasis, the OR were taken from the supplementary data of a published meta-analysis [57] (Supplementary Data 1 ). For rs708686 the OR from the additive model described in the manuscript was utilized. Polygenic risk score calculation A polygenic risk score (PRS) for cholelithiasis in the NIHR-RD data was calculated using Mangrove (version 1.21) ( https://cran.r-project.org/web/packages/Mangrove/index.html ) [63] with the previously published cholelithiasis OR [57] and reference European AF, as described above. The PRS was calculated assuming additivity within and between loci. Statistical comparison of the PRS in cases and controls was performed using an unpaired two-sample two-sided Wilcoxon rank-sum test. Power calculations for the PRS analyses were performed through simulating genotype data for case and control datasets using custom code, written in R (available on request). Genotypes were simulated for each variant in each individual with the probabilities of each genotype status (homozygous reference, heterozygous, and homozygous alternate) determined by the Hardy–Weinberg equilibrium formulae based on the AF and assuming complete linkage equilibrium between the variants. For controls, the reference European AF were used. For cases, the AF of the risk allele were calculated from the reference AF and OR. A total of 100 repetitions of the simulation process were performed in which genotypes for the target variants were generated for the required number of cases and controls (matching the numbers available in the ICP analysis). For each repetition, PRS were generated for each individual using Mangrove, and the statistical significance of the difference between cases and controls was calculated using Wilcoxon rank-sum test. The power to detect a difference was then determined as the percentage of simulations in which a statistically significant difference between cases and controls was seen at P < 0.05. Unbiased gene prioritization and expression/pathway/GWAS Catalog analyses An unbiased assessment of gene expression and functional pathway enrichment of the genes within the 11 prioritized risk loci was undertaken as follows. All 655 variants achieving P < 5 × 10 −8 in the final meta-analysis were identified. Of these, 629 were successfully mapped to an rsID. All variants in LD with these variants at r 2 > 0.8 in European individuals using 1000 Genomes data were identified using LDlinkR (version 1.1.2) ( https://cran.r-project.org/web/packages/LDlinkR/vignettes/LDlinkR.html ) [64] . This resulted in the identification of 871 unique variants. These variants were subsequently analyzed using the Ensembl Variant Effect Predictor (VEP) [65] (version 104) ( https://www.ensembl.org/info/docs/tools/vep/index.html ) to identify the 39 unique genes impacted. These genes were interrogated using the GENE2FUNC tool in FUMA (version 1.3.6b) ( https://fuma.ctglab.nl/gene2func ) [66] . 35 genes were successfully mapped and analyzed by GENE2FUNC ( ABCB1, ABCB11, ABCB4, ABCG5, ABCG8, ATP4A, BABAM2, C2orf16, CCDC121, CRX, CYP7A1, DHRS9, EIF2B4, ENPP7, GAPDHS, GCKR, GPN1, HNF4A, LINC01595, MRPL33, NSMAF, PPIAP85, PPP4R4, RBKS, SBSN, SDCBP, SERPINA1, SERPINA10, SERPINA2, SERPINA6, SHROOM3, SNX17, SULT2A1, TMEM147, TMEM147-AS1, TPRX2P, UBXN2B, ZNF512 , and ZNF513 ). The results of tissue-specificity analysis (as per GTEx [34] data ( https://www.gtexportal.org )), gene sets/pathway analysis (as per MsigDB [67] ( https://www.gsea-msigdb.org/gsea/msigdb )) and overlap of the genes with GWAS Catalog [45] reported associations ( https://www.ebi.ac.uk/gwas/ ) were interrogated. Further details regarding the methodology employed by GENE2FUNC are available on the FUMA website ( https://fuma.ctglab.nl/tutorial#g2fOutputs ). Statistical significance was assessed using hypergeometric tests with Bonferroni correction for multiple testing. Overlap with previous GWAS findings Previously described GWAS findings (as per the GWAS Catalog ( https://www.ebi.ac.uk/gwas ) [45] accessed on July 23, 2021) were searched for overlap with the lead variants at each of the 11 genome-wide significant ICP loci. This was undertaken using the LDtrait Tool from LDlink ( https://ldlink.nci.nih.gov/?tab=ldtrait ) [68] . All associations achieving P < 5 × 10 −6 that were in LD with the 11 identified lead variants at r 2 > 0.6 in European populations (using 1000 Genomes data) were included. Phenotype labels were manually amended such that they were consistent and duplicates were removed (Supplementary Fig. 8 ). Identification of adult human liver replicated accessible regions In order to functionally annotate ICP risk variants, we retrieved from the ENCODE portal [18] ( https://www.encodeproject.org/ ) the IDR ranked peaks for a set of high-quality ATAC-seq experiments carried out on four adult human liver samples. The file identifiers were ENCFF948WBQ, ENCFF012SCX, ENCFF658LHI, and ENCFF658LHI, and corresponded to liver samples from two males and two females with ages ranging from 40 to 61 years old (mean 47 years old). Using these files, we identified the set of genomic regions that were accessible in at least two of the four donors, which we used to prioritize and identify functional ICP regulatory variants. These regions are provided in Supplementary Data 5 (coordinates from genome assembly GRCh38/hg38). Variant functional prioritization The overall prioritization strategy to identify the most likely risk causal variants and genes at each of the ICP-associated loci is presented in Fig. 2 . Details of each of the steps taken to prioritize causal variants and genes are described in the next sections. Statistical fine-mapping We applied PAINTOR (version 3.1) ( https://bogdan.dgsom.ucla.edu/pages/paintor/ ) [17] (a Bayesian fine-mapping approach) which uses an empirical Bayes prior to integrate functional annotation data, LD patterns and strength of association to estimate the posterior probability (PP) of a variant being causal. Variants within a 100-kb window centering on the lead variant at each of the 11 genome-wide significant loci in the meta-analysis were included. LD matrices of pairwise correlation coefficients were derived using European 1000 Genomes (Phase 3) imputed data [69] , excluding variants with ambiguous alleles (A/T or G/C) where reference/alternate alleles could not be reliably matched. Each variant was intersected with the following functional annotations to generate a PP of being causal (PP func ): PhastCons elements (phastConsElements100way, updated August 5, 2015), ENCODE [18] ATAC-seq replicated peaks generated from the adult liver (see above), and Roadmap E066 (adult liver) ChIP-seq narrow peaks for H3K27ac and H3K4me1 histone modifications. Variants with PP func > 0.8 were prioritized for further investigation. For the loci in which PAINTOR did not identify at least one variant with a high posterior probability of being causal (PP func > 0.8), we then proceeded to intersect the coordinates of all ICP variants in the locus with human adult liver accessible chromatin sites (see details above) using pybedtools version 0.8.0 [70] ( https://daler.github.io/pybedtools/ ). This approach was taken because none of the remaining loci contained coding variants. To carry out this analysis, we first defined ICP variants as either (a) all variants within the 95% credible set defined in the ICP GWAS meta-analysis by LocusZoom, or (b) all variants in high LD ( r 2 > 0.8) with the meta-analysis lead variant in European (EUR) individuals. High LD variants were identified using LDlink ( https://ldlink.nci.nih.gov/?tab=ldproxy ). Variant functional annotation of coding variants ICP risk variants were first annotated in relation to their potential to disrupt protein-coding sequences. We identified four ICP-associated loci in which there was at least one coding non-synonymous risk variant. To investigate their potential pathogenicity, we first interrogated them in ClinVar ( https://www.ncbi.nlm.nih.gov/clinvar/ ) [71] . For the ICP coding variants not reported as pathogenic in ClinVar, we performed further pathogenicity analysis using MetaDome [23] (version 1.0.1), which is based on the concept of protein domain homology in the human genome. Briefly, homologous Pfam protein domains were aggregated into meta-domains. Then, population variation from the Exome Aggregation Consortium (ExAC) ( https://exac.broadinstitute.org/ ) and pathogenic mutations from the Human Gene Mutation Database (HGMD) [72] ( http://www.hgmd.cf.ac.uk/ac/index.php ) were used to create genetic tolerance profiles across human meta-domains at amino acid resolution. MetaDome genetic tolerance profiles were previously derived using 56,319 transcripts, 71,419 protein domains, 12,164,292 genetic variants from gnomAD [73] , and 34,076 pathogenic mutations from ClinVar [71] and queried via the online portal at https://stuart.radboudumc.nl/metadome . Interrogation of the coding variant in the GCKR gene was not possible due to a lack of data availability. Finally, we retrieved the CADD scores of pathogenicity (release version 1.6, GRCh38/hg38) for all coding variants from https://cadd.gs.washington.edu/download . The pathogenicity analysis results are presented in Supplementary Data 3 . Analysis of the survey of regulatory elements data Survey of Regulatory Elements was previously performed in HepG2 cells [31] . In that study, the authors interrogated 5.9 million human biallelic SNPs for their ability to confer allele-dependent regulatory activity. We retrieved this dataset (SuRE_SNP_table_LP190708.txt.gz) from https://osf.io/pjxm4/ and queried all ICP variants (see details above) at each of the 11 ICP risk loci. Data are presented as non-risk versus risk allele. 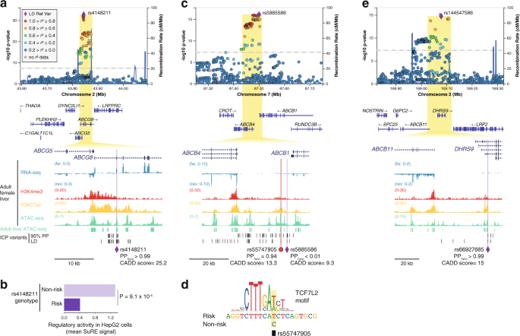Fig. 4: Three ABC transporter gene loci are associated with intrahepatic cholestasis of pregnancy (ICP). a,c,eLocusZoom61plots showing the association signals atABCG8,ABCB1/4, andDHRS9, respectively. The LocusZoom plots are as per Fig.3and association testing was performed as described in Fig.1. At each locus, a single noncoding variant was prioritized as likely causal following the strategy outlined in Fig.2. All epigenomic and transcriptomic datasets shown were retrieved from ENCODE18. Adult liver ATAC-seq peaks track (green regions) corresponds to regions accessible in at least two out of four ENCODE adult liver ATAC-seq (see Methods). 95% PP ICP variants, variants within the 95% genetic credible set in the ICP meta-analysis. LD ICP variants, variants with EURr2> 0.8 with the meta-analysis lead variant. PPfunc, functional posterior probability calculated using PAINTOR17. CADD, combined annotation-dependent depletion.aZoomed inset shows a coding variant atABCG8overlapping a hepatic transcriptional enhancer, as revealed by strong H3K27ac enrichment and accessible chromatin in adult female liver tissue. Metadome analysis did not suggest that this variant affects protein function (see Supplementary Fig.7).bAllele-specific effect of the prioritized risk variant rs4148211, assessed by Survey of Regulatory Elements (SuRE) in HepG2 cells31. The results suggest that the risk variant associates with decreased transcriptional activity. Mean signal and two-sided Wilcoxon rank-sum test. Previously determined 5% false-discovery rate threshold:P< 0.0017312131. Source data are provided as a Source Data file.c,eZoomed insets show two prioritized regulatory risk variants for ICP: one affecting a hepatic enhancer betweenABCB1andABCB4(c), and one affecting a hepatic enhancer in an intron ofDHRS9(d). We note however thatDHRS9is not expressed in liver tissue, as shown in the strand-specific RNA-seq tracks. In contrast,ABCB11is highly expressed in this tissue making it a likely effector transcript in this locus. P values were obtained by a two-sided Wilcoxon rank-sum test, comparing for each SNP the set of SuRE values of all fragments containing the reference allele versus the set of SuRE values of all fragments containing the alternative allele. 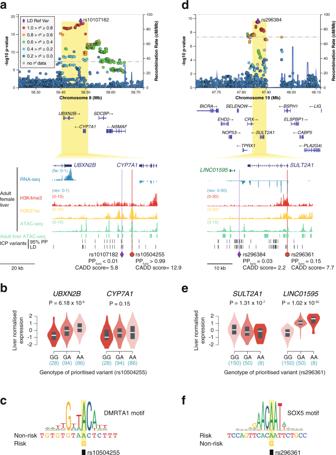Fig. 5: GWAS meta-analysis of ICP reveals association signals affecting the bile acid homeostasis genesCYP7A1andSULT2A1. a,dLocusZoom61plots showing the association signals atCYP7A1andSULT2A1, respectively. The LocusZoom plots are as per Fig.3and association testing was performed as described in Fig.1. All epigenomic and transcriptomic datasets shown were retrieved from ENCODE18. Adult liver ATAC-seq peaks track (green regions) corresponds to regions accessible in at least two out of four ENCODE adult liver ATAC-seq (see “Methods”). 95% PP ICP variants, variants within the 95% genetic credible set in the ICP meta-analysis. LD ICP variants, variants with EURr2> 0.8 with the meta-analysis lead variant. PPfunc, functional posterior probability calculated using PAINTOR. CADD, combined annotation-dependent depletion.aFunctional fine-mapping with PAINTOR17identified a single variant (rs10504255) with a posterior probability over 0.99 overlapping an active liver enhancer located between theCYP7A1gene, which encodes the rate-limiting enzyme for bile acid synthesis, andUBXN2B.b,eGTEx34[GTEx Analysis Release V8 (dbGaP Accession phs000424.v8.p2)] human liver eQTLs identify the top prioritized variant in theCYP7A1locus (rs10504255) as an eQTL associated with the eGeneUBXN2B(b) and show that theSULT2A1promoter ICP variant (rs296361) is an eQTL for bothSULT2A1and its downstream lncRNALINC01595(e). Violin plots represent the density distribution of the samples in each genotype (nfor each genotype is indicated below in blue). Box plots show normalized gene expression in median (white line), first and third quartiles. Gene-level adjustedPvalues calculated with FastQTL85are shown.cThe risk allele of the ICP-associated variant rs10504255 (G) disrupts a DMRTA1-binding motif. We note that this allele also associates with weaker transactivation in liver tissue, as observed by eQTL analysis (b).dOverlap of ICP risk variants with adult liver accessible chromatin sites revealed one variant in the promoter ofSULT2A1(rs296361).fTranscription factor motif analysis revealed that the ICP variant rs296361 affects a motif for the SOX-D transcriptional repressor family. Following the original report [31] , P < 0.00173121 were considered as passing a 5% false-discovery rate threshold. Data mining was performed using Python (version 3.7) and figures were plotted using seaborn [74] version 0.11.2 ( https://seaborn.pydata.org/ ). Transcription factor binding motif analysis The prioritized ICP-associated variants (see details above) were investigated for their potential effect on TF binding affinity using Motifbreak R version 2.2.0 ( https://bioconductor.org/packages/release/bioc/html/motifbreakR.html ). To query motifs, we imported MotifDb ( https://bioconductor.org/packages/release/bioc/html/MotifDb.html ) (version 1.30.0), which contains >4200 TF motifs, including >2800 motifs from studies in human samples and includes the databases HOCOMOCO [75] , HOMER [76] , and ENCODE-motifs [18] . For visual representation, motif logos were downloaded from JASPAR 2020 [77] ( http://jaspar.genereg.net/ ). Analysis of human liver eQTLs Human liver eQTL data shown in this study were retrieved from the Genotype-Tissue Expression (GTEx) Portal [34] on May 12, 2021, which at the time of accession contained data for 208 liver samples. [GTEx Analysis Release version 8 (dbGaP Accession phs000424.v8.p2)]. At each ICP association signal, we queried the lead variant and, if different, the variant that was functionally prioritized. The analysis was restricted to liver eQTLs and eGenes contained in the same TAD as the lead variant (human liver TAD coordinates were retrieved from http://3dgenome.fsm.northwestern.edu/publications.html ). Figures were directly downloaded from the GTEx Portal. Analysis of adult liver 3D chromatin conformation Gene expression and eQTL analyses were restricted to the topologically associating domains (TADs) containing the ICP-associated variants identified in our meta-analysis. Human liver TAD coordinates (GRCh38/hg38) [78] were retrieved from http://3dgenome.fsm.northwestern.edu/downloads/hg38.TADs.zip . 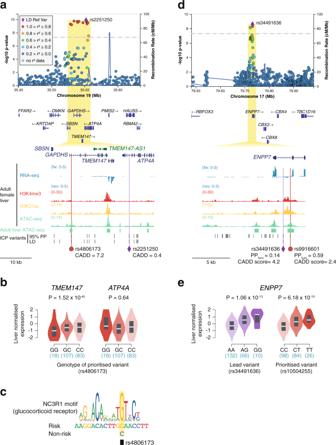Fig. 6: Analysis human liver eQTLs uncoversTMEM147andENPP7as effector transcripts of ICP susceptibility. a,dLocusZoom86plots showing the association signals atTMEM147andENPP7, respectively. The LocusZoom plots are as per Fig.3and association testing was performed as described in Fig.1. All epigenomic and transcriptomic datasets shown were retrieved from ENCODE18. Adult liver ATAC-seq peaks track (green regions) corresponds to regions accessible in at least two out of four ENCODE adult liver ATAC-seq (see “Methods”). 95% PP ICP variants, variants within the 95% genetic credible set in the ICP meta-analysis. LD ICP variants, variants with EURr2> 0.8 with the meta-analysis lead variant. PPfunc, functional posterior probability calculated using PAINTOR17. CADD, combined annotation-dependent depletion. Overlap of ICP-associated variants in these two loci with adult liver accessible chromatin sites enabled the prioritization of two ICP regulatory variants in intronic regions ofGAPDHS(rs4806173) (a) andENPP7(rs9916601) (d).b,eThe ICP variants prioritized with functional liver chromatin annotations are eQTLs in liver tissue and pinpointTMEM147andENPP7as effector transcripts in these loci. Violin plots represent the density distribution of the samples in each genotype (nfor each genotype is indicated below in blue). Box plots show normalized gene expression in median (white line), first and third quartiles. Gene-level adjustedPvalues calculated with FastQTL86are shown. Liver eQTL plots were retrieved from GTEx34[GTEx Analysis Release V8 (dbGaP Accession phs000424.v8.p2)]. We note thatGAPDHSis a testis-specific gene and its interrogation as an eGene for rs4806173 was therefore not possible (b).cThe ICP risk allele of rs4806173 (G), which associates with less transcription ofTMEM147, is predicted to create a binding site for glucocorticoid receptors, a family of context-dependent transcriptional regulators that can act as either activators or repressors87. 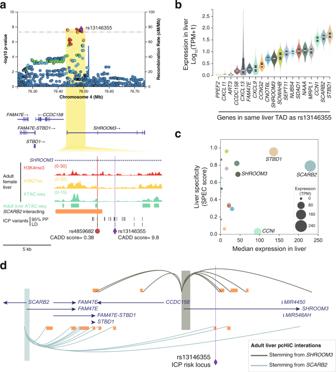Fig. 7: Tissue-specificity and 3D chromatin conformation analyses prioritize SCARB2 as an ICP susceptibility gene. aLocusZoom86plot showing the association signal atSHROOM3. The LocusZoom plots are as per Fig.3and association testing was performed as described in Fig.1. All epigenomic and transcriptomic datasets shown were retrieved from ENCODE18. Adult liver ATAC-seq peaks track (green regions) corresponds to regions accessible in at least two out of four ENCODE adult liver ATAC-seq (see “Methods”). 95% PP ICP variants, variants within the 95% genetic credible set in the ICP meta-analysis. LD ICP variants, variants with EURr2> 0.8 with the meta-analysis lead variant. CADD, combined annotation-dependent depletion. Overlap of ICP risk variants in this locus with adult liver accessible chromatin sites enabled the prioritization of a single ICP-regulatory variant in an intronic region of theSHROOM3gene (rs4859682). None of the other ICP variants (EURr2> 0.8 with lead variant or in the 95% PP credible set) overlapped accessible chromatin sites.bExpression of all genes within the TAD containing the ICP lead variant rs13146355 in the human liver. Expression data was retrieved from GTEx34[GTEx Analysis Release V8 (dbGaP Accession phs000424.v8.p2)]. Violin plots represent the density distribution of expression of the indicated genes in human liver tissue (n= 226 donors). Box plots show gene expression in median (white line), first and third quartiles. TPM, transcripts per million. Note that the gene harboring the ICP risk variant,SHROOM3, is lowly expressed in the liver.cScatter plot showing the expression of all genes within the TAD containing the ICP lead variant rs13146355 in the human liver versus their liver-specificity. Tissue-specificity scores (SPECS) were precalculated by Everaert et al.81. Source data are provided as a Source Data file. This plot highlights two highly expressed and liver-specific genes,STBD1,andSCARB2.d, Analysis of long-range chromatin interactions in human liver detected by promoter capture Hi-C79, showing that the genomic region containing the ICP risk variant rs4859682 interacts withSCARB2, but notSHROOM3. Long-range chromatin interactions stemming from the promoter ofSTBD1were not detected in liver tissue. For specific investigation of long-range chromatin interactions in liver tissue, we interrogated two complementary datasets from adult liver: Hi-C [78] and capture Hi-C [79] . These datasets were visualized and analyzed using the 3D-genome interaction viewer and database ( http://www.3div.kr/ ). Visualization of human adult liver datasets Human adult female liver (right lobe) epigenomic and transcriptomic datasets we downloaded from the ENCODE portal [18] ( https://www.encodeproject.org/ ) in bigwig format and visualized using the UCSC Genome Browser [80] (GRCh38/hg38). All data corresponds to fold change over control for the shown assay. The visualized files had the following identifiers: ENCFF232QBB (ATAC-seq), ENCFF280QYJ (H3K4me3 ChIP-seq) and ENCFF853WPX (H3K27ac ChIP-seq). Adult liver 3D chromatin interaction datasets were visualized and analyzed using the 3D-genome interaction viewer and database ( http://www.3div.kr/ ). Tissue-specificity analysis In order to investigate whether the ICP risk variants at SHROOM3 could be in the vicinity of or interact with liver-specific genes, we used SPECS scores [81] , which were pre-computed for adult liver for all Ensembl (GRCh38.v85) genes using all GTEx [34] samples. In brief, SPECS is a non-parametric tissue-specificity score that is compatible with unequal sample group sizes. SPECS uses all individual data points available and enables the detection of features that are specifically present or absent in one or more tissue types. The SPECS score has been shown to outperform other tissue-specificity scores [81] , including z-score [82] and JSD [83] . Data mining was performed using Python (v3.7) and figures were plotted using seaborn [74] version 0.11.2 ( https://seaborn.pydata.org/ ) [18] . Reporting summary Further information on research design is available in the Nature Research Reporting Summary linked to this article.